The importance of stress percolation patterns in rocks and other polycrystalline materials A new framework for thinking about the deformation behavior of rocks and other heterogeneous polycrystalline materials is proposed, based on understanding the patterns of stress transmission through these materials. Here, using finite element models, I show that stress percolates through polycrystalline materials that have heterogeneous elastic and plastic properties of the same order as those found in rocks. The pattern of stress percolation is related to the degree of heterogeneity in and statistical distribution of the elastic and plastic properties of the constituent grains in the aggregate. The development of these stress patterns leads directly to shear localization, and their existence provides insight into the formation of rhythmic features such as compositional banding and foliation in rocks that are reacting or dissolving while being deformed. In addition, this framework provides a foundation for understanding and predicting the macroscopic rheology of polycrystalline materials based on single-crystal elastic and plastic mechanical properties. One of the hallmark features of deformed rocks is the presence of patterns; for example, patterns created by shear localization, patterns associated with preferential dissolution like stylolites and slatey cleavage or patterns such as compositional banding that are created by mineral segregation. Even rocks that appear initially homogeneous like shale or randomly patterned like granites develop patterned features when deformed in the Earth’s interior. A question that has puzzled many geologists is: how and why do these patterns arise? The role of stress in governing the orientation of features has long been recognized—stylolites, foliation and compositional banding form perpendicular to compression, fractures form at 30° to compression and shear zones at 45°. But what governs their spacing? What causes them to arise from an unpatterned material? Much research has been done on each type of feature separately but there is no overarching theory for pattern formation in deformed rocks. The behavior of any given crystal within a polycrystalline material is governed by its intrinsic response to the boundary conditions imposed upon it; lattice scale processes that are easily observed and relatively well understood (for example, fracture, dislocation slip and climb/cross slip, twinning and diffusion creep). What is not easily understood is how the boundary conditions applied to each crystal relate to the boundary conditions placed upon the aggregate. If the grains in a rock or polycrystalline aggregate have identical responses to loading then there is no reason to suspect that local boundary conditions should differ from those at the exterior boundary. However, for aggregates with elastic and plastic anisotropy, various grain populations will respond to stress differently. Thus, the boundary conditions imposed upon any given grain are moderated by the responses of its neighbors and in turn by its neighbors’ neighbors. Researchers have attempted to understand the effect of a grain’s neighborhood by modeling small ensembles of grains and examining the impact of changing the properties of a grain’s neighbors [1] , [2] , [3] , [4] , [5] . However, especially for highly anisotropic materials like minerals, there is little to guide us in determining how large the ensemble or so-called ‘representative volume element’ (RVE) needs to be to capture the full variety of mechanical situations that arise within the aggregate. This study was motivated by a desire to understand how bulk rheology relates to the mechanical behavior of a material’s constituent crystals, but the results serve as a framework for thinking about all pattern formation in deformed rocks. In order to determine if long-range or short-range interactions are important for stress heterogeneity, I have used two-dimensional (2D) plane-strain finite element models of a large ensemble of grains in a hypothetical elastic–plastic polycrystalline material. The grains are divided into 25 subsets to which mechanical properties are assigned. No motion between the grains is permitted on the grain boundaries, thus grain boundaries are demarcated only by a change in elastic and plastic properties. When the models are compressed, large-scale patterns in the local stress tensor arise. The density of the patterning is dictated by the degree of heterogeneity in and statistical distribution of the elastic and plastic properties of the grains. The stress patterning and the patterns of shear localization that arise once plastic deformation initiates are described below. Results of finite element models All models with heterogeneities in the mechanical properties show large-scale patterns of stress maxima and minima when they are compressed. The arrangement of grains in the models is illustrated in Fig. 1 . The nature of the patterns in stress and how the patterns are impacted by elastic heterogeneity is illustrated in Fig. 2 , which shows the equivalent von Mises stress for four of the models. In all models illustrated here, compression is in the vertical direction. In Fig. 2a the Young’s moduli of the grains varies from 0 to 500 GPa. Although this degree of variation in elastic properties is unrealistic, I use this model as an extreme end-member. In Fig. 2d the Young’s moduli of the grains varies from 100 to 120 GPa, which is similar to the degree of variation seen in high-symmetry minerals like beta quartz or halite. 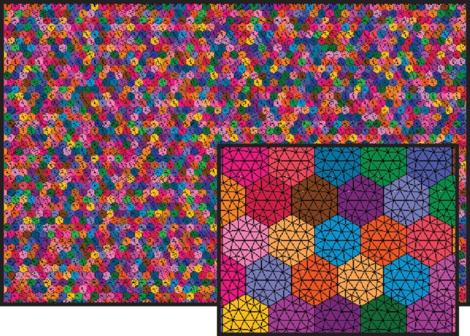Figure 1: Finite element model used in this study. The inset shows an enlarged region of the mesh. The hexagonal grains are color-coded by grain set. Rheological properties are assigned to each grain set. The other models have variations in elastic properties that are intermediate ( Table 1 ). Although the patterns occur on a scale much larger than the grain-scale, they do not reflect the pattern of grain boundaries because individual grains contain significant stress gradients. In Fig. 2d the pattern can be described as isolated islands of low equivalent stress, but in Fig. 2a one can see braided ‘streams’ of high equivalent stress running vertically through the models. The change in patterning from the most heterogeneous model to the least is in the spacing of the ‘streams’ and the intensity of the stress concentration in the ‘streams’. The vertically oriented patterns originate from variations in the magnitude and direction of the maximum compressive stress ( σ 3 ). A subordinate horizontal pattern (best seen in Fig. 2a ), results from variations in σ 1 . Figure 3 shows a portion of a model with the full stress tensor plotted. 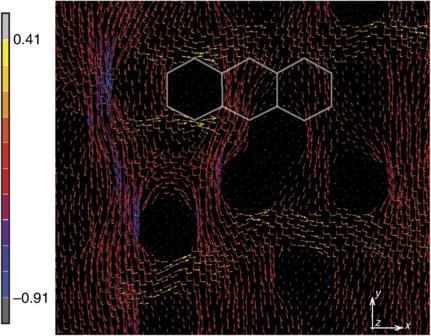Figure 3: Local variations in the stress tensor within model hex16. Orientation and magnitude of minimum (σ3) and maximum (σ1) components of the stress tensor in a portion of model hex16. Compression (which is negative), is depicted in orange to blue; tensile stresses are yellow. The arrows point in the direction of the principal components of the tensor. The position and size of three grains is outlined in gray for scale. With the exception of the softest grains, the patterns of stress magnitude and orientation largely ignore the identity of the grains. The orientation of the maximum compressive stress can deviate substantially away from the macroscopic compression direction and the stress state can even become tensile. These variations are produced by the difference in elastic properties of neighboring grains even before plastic flow in the weakest grains initiates. The patterns in stress are established in the first displacement increment and change only in numerical value until the first yielding occurs. As yielding initiates, the patterning in σ 3 deteriorates, while the patterning in σ 1 intensifies ( Fig. 4 ). All of the models produce strain localization in the form of shear bands ( Fig. 5 ), and the spacing of the shear bands is coupled to the stress patterning; denser patterning produces more closely spaced shear bands concentrating smaller degrees of stain. Shear localization develops at very low strains and intensifies between locations where yielding initiates. Therefore, the location of shear bands is dictated by the spatial distribution of locations where yielding first occurs ( Fig. 6 ). The degree to which shear bands grow and intensify or not as a function of global strain depends on the level of work hardening included in the plasticity model. Figure 1: Finite element model used in this study. The inset shows an enlarged region of the mesh. The hexagonal grains are color-coded by grain set. 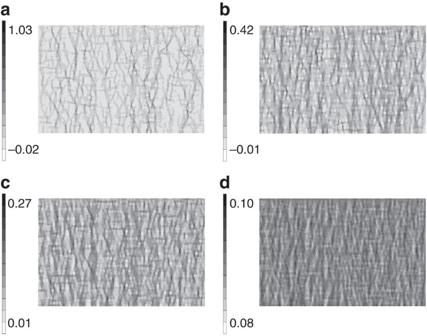Rheological properties are assigned to each grain set. Figure 2: Equivalent von Mises stress patterns. Equivalent von Mises stress patterns for models with a variety of elastic properties. Dark shades are higher values and light shades are for lower values. A compressional load of 0.1 GPa in the vertical direction was used. (a) Grains withE=500 to 0 GPa andv=0.1 to 0.4 (model hex20), (b) grains withE=500 to 0 GPa andv=0.3 (model hex16), (c) grains withE=200 to 20 GPa andv=0.3 (Model hex9) and (d) grains withE=120 to 100 GPa andv=0.3 (Model hex18). The maximum value of the equivalent stress in hex20 is 10 times that found in hex18. Full size image Figure 2: Equivalent von Mises stress patterns. Equivalent von Mises stress patterns for models with a variety of elastic properties. Dark shades are higher values and light shades are for lower values. A compressional load of 0.1 GPa in the vertical direction was used. ( a ) Grains with E =500 to 0 GPa and v =0.1 to 0.4 (model hex20), ( b ) grains with E =500 to 0 GPa and v =0.3 (model hex16), ( c ) grains with E =200 to 20 GPa and v =0.3 (Model hex9) and ( d ) grains with E =120 to 100 GPa and v =0.3 (Model hex18). The maximum value of the equivalent stress in hex20 is 10 times that found in hex18. Full size image Table 1 Mechanical properties of grain sets in models used for illustrations. Full size table Figure 3: Local variations in the stress tensor within model hex16. Orientation and magnitude of minimum ( σ 3 ) and maximum ( σ 1 ) components of the stress tensor in a portion of model hex16. Compression (which is negative), is depicted in orange to blue; tensile stresses are yellow. The arrows point in the direction of the principal components of the tensor. The position and size of three grains is outlined in gray for scale. 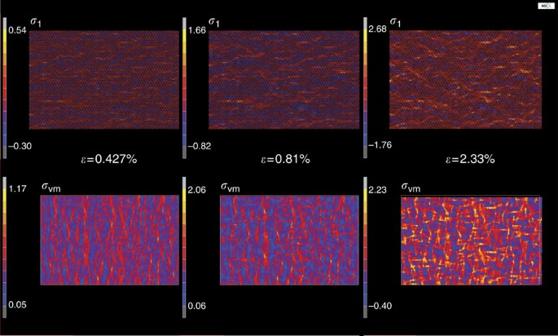Figure 4: Changes in stress tensor patterns during yielding. Patterns inσ1and equivalent von Mises stress (σvm) for model hex9 prior to (0.47% strain), during (0.81% strain) and after (2.33% strain) yielding initiates. This model has no work hardening. The patterns inσ1intensify as grains in the model begin to deform plastically, which causes the patterns inσvmto become less coherent. Full size image Figure 4: Changes in stress tensor patterns during yielding. Patterns in σ 1 and equivalent von Mises stress ( σ vm ) for model hex9 prior to (0.47% strain), during (0.81% strain) and after (2.33% strain) yielding initiates. This model has no work hardening. The patterns in σ 1 intensify as grains in the model begin to deform plastically, which causes the patterns in σ vm to become less coherent. 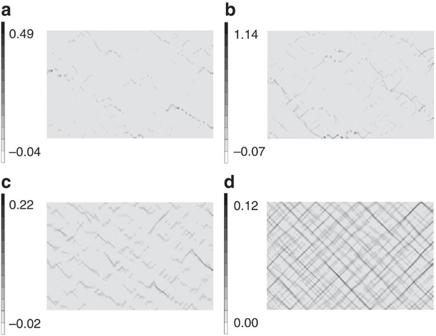Figure 5: Patterns in equivalent plastic strain. Patterns in equivalent plastic strain for models shown inFig. 2. Dark shades are higher values and light shades are lower values of equivalent plastic strain. Models are shown at a strain increment between 0.2–0.5% global strain beyond initial yielding. (a) hex20, (b) hex16, (c) hex9 and (d) hex18. Full size image Figure 5: Patterns in equivalent plastic strain. Patterns in equivalent plastic strain for models shown in Fig. 2 . Dark shades are higher values and light shades are lower values of equivalent plastic strain. Models are shown at a strain increment between 0.2–0.5% global strain beyond initial yielding. ( a ) hex20, ( b ) hex16, ( c ) hex9 and ( d ) hex18. 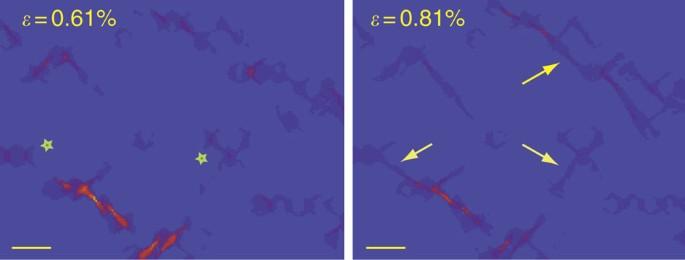Figure 6: Changes in equivalent plastic strain during shear localization. Plot of equivalent plastic strain for a portion of model hex9. Scale bar is equivalent to the width of two grains. Most grains exhibit no plastic strain (purple). Grains where yielding initiates (deep purple to orange) develop ‘fins’ that extend outwards at 45° (green stars). Fins connect between grains when yielding grains are sufficiently close (yellow arrows). Full size image Figure 6: Changes in equivalent plastic strain during shear localization. Plot of equivalent plastic strain for a portion of model hex9. Scale bar is equivalent to the width of two grains. Most grains exhibit no plastic strain (purple). Grains where yielding initiates (deep purple to orange) develop ‘fins’ that extend outwards at 45° (green stars). Fins connect between grains when yielding grains are sufficiently close (yellow arrows). Full size image The FEM models presented here make predictions about the heterogeneity and spatial distribution of elastic and plastic strain in polycrystalline materials that are consistent with experimental observations as well as results from other numerical studies. Many microstructural studies of plastically deformed polycrystals observe intragranular heterogeneity of plastic strain ranging from those conducted on highly anisotropic materials like olivine and ice [6] , [7] to metals, which generally have more isotropic single-crystal rheological properties [2] , [8] , [9] , [10] , [11] . The degree of strain heterogeneity is thought to be a function of the anisotropy of the material [1] , [7] . The development of shear-strain localization at very low degrees of strain has been observed in a number of materials [7] , [8] , [11] , [12] . The development of tensile elastic strain during compression has been observed in ice [7] and zirconium [11] . Large variations in stress states within single grains and plastic features that span many grains have been observed in three-dimensional (3D) finite element models of polycrystalline FCC metals [1] . However, consistent with what is observed in synchrotron and neutron diffraction studies of deforming materials, elastically stiffer grains on average strain less than more compliant grains (see, for example, the study by Turner and Tome [13] , or diffraction data within the study by Burnley and Zhang [14] ) ( Fig. 7 ). 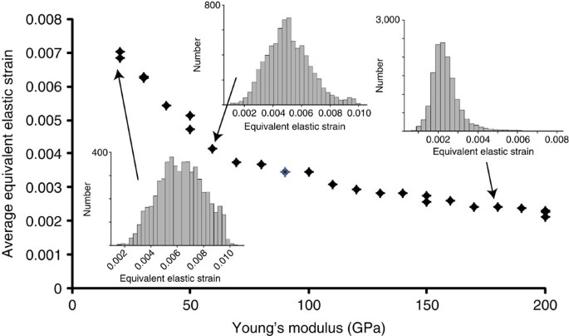Figure 7: Average equivalent elastic strain versus Young’s modulus. Average equivalent elastic strain for nodes in grain sets as a function of the Young’s modulus assigned to each grain set in model hex9 at 0.12% shortening. Histograms showing the distribution of equivalent elastic strain across the nodes in each of three grain sets (materials 10, 1 and 20) are given as insets. Figure 7: Average equivalent elastic strain versus Young’s modulus. Average equivalent elastic strain for nodes in grain sets as a function of the Young’s modulus assigned to each grain set in model hex9 at 0.12% shortening. Histograms showing the distribution of equivalent elastic strain across the nodes in each of three grain sets (materials 10, 1 and 20) are given as insets. Full size image Large-scale patterning of stress in granular materials is well known [15] , [16] , [17] , [18] , [19] . Referred to as force chains, the patterns are produced by stress percolation [20] and consist of semi-linear subsets of particles arranged parallel to compression that bear the applied load through the so-called ‘strong’ contacts between them. Granular materials are most obviously distinct from fully dense polycrystalline materials in that the constituent grains have limited or no cohesion. Both shear tractions and tensile forces are strongly or entirely dissipated on grain boundaries. In granular materials there are extreme variations in the mechanical properties of the constituent structural components (grain boundaries and grain interiors), whereas in fully dense polycrystalline materials variations between structural components, which may or may not include rheologically distinct grain boundaries [21] , are comparatively muted. Thus, granular materials and fully dense polycrystalline materials fall on a continuum of variation in component properties. The value in making this connection is that it suggests new ways of thinking about deformation of polycrystalline materials. For example, force chains are understood to be the underlying mechanism of shear localization in granular materials (see Discussion in the study by Tordesilla and Muthuswamy [22] and references therein). Therefore, examining the role of stress patterning in shear localization in polycrystalline materials may prove fruitful. The magnitude of stress concentrations in the stress patterns and the regularity with which they occur may well yield to statistical descriptions, as they do in granular materials [23] and should lead to a better understanding of phenomena that are tied to stress concentrations, such as the development of stylolites, slatey cleavage and compositional banding in rocks [24] , [25] , as well as help explain how these rhythmic features initially arise from unpatterened rocks such as shale and granite. The recognition of stress patterning will have a number of important implications for experimental characterization and modeling of rheological properties. In experimental studies, the scale of stress patterning dictates the size of the RVE needed for testing. Experimental samples whose size allows only a portion of the stress pattern to be captured, may present difficulties for obtaining reproducible results; a phenomena that would be most noticeable in high-pressure studies where sample sizes are restricted. Changing the grain size or overall size of experimental samples can be cumbersome, but numerically it should be comparatively painless to predict the appropriate RVE by increasing the size of the grain ensemble being modeled until the tails of the stress distribution are fully described. Another important implication of stress patterning is that it provides a framework for modeling aggregate behavior over multiple-length scales based on single-crystal properties. Robust predictive models of the mechanical behavior of rocks are needed for understanding the mechanical behavior of the interior of the Earth and other planets because extrapolations in both length scale and strain rate will always be required [26] . The need for reliable predictive rheological models is not confined to the geosciences but extends to engineering and materials science problems that present a variety of challenges for direct observation; for example, shock loading of nuclear weapon components or detonation of plastic-bonded explosives. These extrapolations can be made with more confidence if they are generated by models that are based on the physics of deformation: capturing the behavior of the crystal lattice as well as the short- and long-range interaction between grains within the polycrystal. So, for example, elastic–plastic and viscoplastic self-consistent models describe single-crystal plasticity but assume that a single set of average boundary conditions apply to each grain. These models could be modified such that the boundary conditions applied to each grain are allowed to vary over a range suitable to the elastic and plastic heterogeneity of the structural components of the material. Perhaps the most important impact that the recognition of stress patterning can have is if it, as a simple and intuitive paradigm, can replace the default assumption of a Reuss state (isostate) of stress in the minds of those who work on stress-related phenomena. Although it has been long recognized that the Reuss state of stress is an oversimplification, the assumption still pervades our thinking on everything from the attenuation of seismic waves to the development of paleopiezometers. By providing a means of leaving the Reuss stress state assumption behind, the recognition of patterning in stress should lead to new insights in a number of disciplines. Finite element models The finite element models were constructed using MSC. MARC/Mentat, a commercial finite element analysis package. Each grain was modeled as a hexagon containing 48 six-noded triangular elements ( Fig. 1 ); this type of element uses a parabolic interpolation function along each edge. The models were calculated assuming a 2D plane-strain geometry utilizing full integration. The nodes on the boundaries of each grain are shared with the elements along the edge of the neighboring grain, thus grain boundaries are demarcated only by a change in elastic and plastic properties. As there can be no offset along a grain boundary in the model, the grain boundaries do not have separate mechanical properties. The model consists of 2,574 hexagonal grains that have been assigned randomly into 25 subsets. All materials used in the model assumed an isotropic linear elastic response. The constitutive equation used for linear elastic solids is: where σ ij is the stress tensor, δ ij is the Kronecker delta, ε ij is the strain tensor, λ is the Lame constant, and G is the shear modulus. λ can be expressed as: and G can be expressed as: where v is the Poisson’s ratio and E is the Young’s modulus. MARC accepts E and v as inputs to define a material’s elastic properties. Plastic behavior initiates when the equivalent von Mises stress ( σ vm ), which is calculated as follows: equals the specified yield strength. Post-yielding behavior was either perfectly plastic or included a work-hardening slope. The Young’s modulus and Poisson’s ratio assigned to each grain set for the models presented in the illustrations are given in Table 1 . For all materials shown in the figures, the yield strength was set to 1/100th of the Young’s modulus and no work hardening was included. Boundary conditions were applied along three edges of the models. Nodes along the bottom edge were not allowed to move in y (the vertical axis). Nodes along the left edge were not allowed to move in x (the horizontal axis). Depending on the goal of the experiment, either a constant edge load was placed on the top edge of the model or a constant displacement was applied to each node on the top of the model. The right edge of each model was allowed to move freely. How to cite this article: Burnley, P. C. The importance of stress percolation patterns in rocks and other polycrystalline materials. Nat. Commun. 4:2117 doi: 10.1038/ncomms3117 (2013).